KCNE1 divides the voltage sensor movement in KCNQ1/KCNE1 channels into two steps The functional properties of KCNQ1 channels are highly dependent on associated KCNE-β subunits. Mutations in KCNQ1 or KCNE subunits can cause congenital channelopathies, such as deafness, cardiac arrhythmias and epilepsy. The mechanism by which KCNE1-β subunits slow the kinetics of KCNQ1 channels is a matter of current controversy. Here we show that KCNQ1/KCNE1 channel activation occurs in two steps: first, mutually independent voltage sensor movements in the four KCNQ1 subunits generate the main gating charge movement and underlie the initial delay in the activation time course of KCNQ1/KCNE1 currents. Second, a slower and concerted conformational change of all four voltage sensors and the gate, which opens the KCNQ1/KCNE1 channel. Our data show that KCNE1 divides the voltage sensor movement into two steps with widely different voltage dependences and kinetics. The two voltage sensor steps in KCNQ1/KCNE1 channels can be pharmacologically isolated and further separated by a disease-causing mutation. Voltage-gated potassium channels (Kv) regulate the membrane potential of excitable cells, controlling the firing and duration of action potentials [1] . Regulatory β-subunits associate with Kv channels to modulate the gating properties of Kv channels [2] . KCNQ1 (Kv7.1 or KvLQT1) is expressed in many different tissues, such as the inner ear, the kidney and the heart [3] . KCNQ1 channels function differently in these tissues, and it is thought that these functional differences are mainly because of association with different types of KCNE β-subunits [3] . Mutations in KCNQ1 or KCNE subunits cause congenital channelopathies, such as deafness, cardiac arrhythmias and epilepsy [4] , [5] , [6] . The KCNQ1 α-subunit expressed alone forms functional tetrameric Kv that open at negative voltages with a time constant of 100 ms (ref. 7 ). Co-assembly of KCNQ1 with KCNE1 slows the activation kinetics and shifts the voltage dependence of KCNQ1 to positive voltages [8] , [9] . KCNE1 also increases the KCNQ1/KCNE1 channel macroscopic current and single-channel conductance compared with KCNQ1 alone [10] . The slow activation kinetics of the KCNQ1/KCNE1 channel critically contributes to its physiological function in the heart by delaying its repolarizing current and thus the termination of the action potential. Contradicting models have been proposed for the mechanism by which KCNE1 affects the activation kinetics of KCNQ1/KCNE1 channels [11] , [12] , [13] , [14] . Using a number of independent methods, we here resolve these contradictions by investigating how KCNE1 affects the activation kinetics of KCNQ1/KCNE1 channels. Like other Kv channels, KCNQ1 has six transmembrane segments (S1–S6) and forms tetrameric channels with a central pore domain (composed of S5–S6) and four peripheral voltage-sensing domains (composed of S1–S4) [15] . The pore domain comprises the K + conduction pathway with the activation gate (S6). Mutations of positively charged residues in the fourth transmembrane domain (S4) in KCNQ1 strongly alter or abolish voltage gating, supporting the notion that S4 acts as the voltage sensor in KCNQ1 channels [16] . Upon depolarization, outward motion of S4 in each subunit mediates voltage sensing and is assumed to open the S6 gate and allow potassium permeation. However, how the voltage sensor movement couples to the opening of the gate is still debated. It is also not clear how the KCNE1 β-subunit affects the KCNQ1 α-subunit. Disulphide crosslinking studies suggested that KCNE1 is located between the voltage sensor domain and the pore domain of KCNQ1, a position where it could affect both the voltage sensor and the activation gate [11] , [17] , [18] , [19] . One cysteine accessibility study showed that KCNE1 slows the modification rate of cysteines introduced in S4 of KCNQ1 to externally applied cysteine reagents [11] . This was interpreted as KCNE1 slowing the outward movement of S4 in response to depolarizing voltage pulses [11] . However, another cysteine accessibility study showed that the modification rate in KCNQ1/KCNE1 channels was independent of the length of depolarizing voltage pulses for durations ≥100 ms, as long as the total time spent depolarized was constant [14] . This suggests that S4 moves out in <100 ms. Because 100 ms is much shorter than the time to open a KCNQ1/KCNE1 channel, the authors concluded that KCNE1 slows the opening of the gate [14] . Using voltage clamp fluorometry (VCF), which simultaneously assesses voltage sensor movement (fluorescence) and channel opening (ionic current), we previously showed that the time courses of the fluorescence and current in KCNQ1 channels alone are similar, but that the time course of fluorescence is much faster than the activation of the currents in KCNQ1/KCNE1 channels [13] . This suggests that KCNE1 mainly slows the gate in KCNQ1/KCNE1 channels [13] . Recently, another VCF study [12] concluded that KCNE1 slows the voltage sensor movement of KCNQ1/KCNE1 channels, but not the gate, because in their experiments the time course of the fluorescence and the ionic current from KCNQ1/KCNE1 channels had similar slow kinetics in the voltage range assayed. In addition, they resolved gating currents in KCNQ1 channels in the absence, but not in the presence, of KCNE1, which is consistent with their conclusion that the gating charge movement is very slow in the presence of KCNE1 (ref. 12 ). From these contradicting studies, it is not clear how KCNE1 affects KCNQ1 channels. In our previous VCF study, the fluorescence from a fluorophore attached to the external end of S4 in KCNQ1/KCNE1 channels displayed two fluorescence components [13] . However, in the light of the more recent VCF study [12] , the origin of these two fluorescence components and how they are coupled to gating charge movement of S4 and channel opening is now controversial. In VCF, it is assumed that changes in fluorescence from the fluorophore attached to a protein segment reports on conformational changes of the protein segments, or a nearby region, that alters the environment around the fluorophore and thereby changes the fluorescence. We assumed that the fast fluorescence component at negative voltages that clearly precedes channel opening was because of S4 gating charge movement [13] . The origin of the second fluorescence component at positive voltages was not clear in our study [13] , and in the study by Ruscic et al. [12] , who only detected the fluorescence component at positive voltages, the fluorescence component at positive voltages was assumed to be because of S4 gating charge movement. We will here investigate the origin of the two fluorescence components and determine how they are coupled to gating charge movement of S4 and channel opening in KCNQ1/KCNE1 channels. Here we use two independent methods (VCF and cysteine accessibility) to show that KCNE1 separates the voltage sensor movement of KCNQ1 into two components. The first component occurs at negative potentials and involves relatively rapid voltage sensor movements. The second component occurs at positive potentials and involves slower voltage sensor movements. The first component generates the main gating charge movement and is reflected in the characteristic delay of the activation time course of the KCNQ1/KCNE1 currents, whereas the second component involves an additional voltage sensor movement simultaneous with channel opening. KCNE1 splits the fluorescence into two components To measure the voltage sensor movement in KCNQ1/KCNE1 channels using VCF, a cysteine introduced at position 219 in the S3–S4 extracellular loop of KCNQ1 is labelled with the fluorophore Alexa488-maleimide [13] . 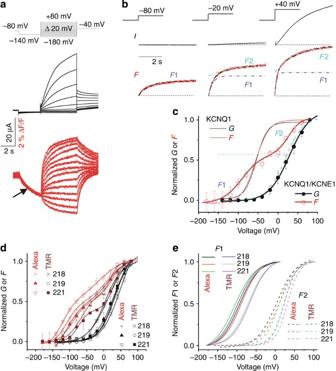Figure 1: KCNE1 splits the voltage sensors movement of KCNQ1 into two components. (a) Representative current (black) and fluorescence (red) traces from KCNQ1/KCNE1 channels for the indicated voltage protocol (top). (b) Current (black) and fluorescence (red) in response to indicated test potentials for 5 s from −140 mV. The fluorescence traces are fit by a single exponential curve for the −80-mV step and a double exponential curve for the steps to −20 mV and +40 mV (black dashed line). The fast (purple dashed-dotted lines) and slow (cyan dashed-dotted lines) exponential curves of the double exponential fits are shown separately, overlaying the early and late part of the data, respectively. (c) NormalizedG(V)(filled black circle and black line from a Boltzmann fit) andF(V)(open red circle and red line from a double Boltzmann fit) of recordings from KCNQ1/KCNE1 channels. The first (purple dashed-dotted lines) and the second (cyan dashed-dotted lines) Boltzmann curves of the double Boltzmann fits are shown separately, overlaying the data at negative and positive voltages, respectively. Data are mean±s.e.m.;n=7. Cyan dashed line represents the second fluorescence component normalized between 0 and 1 for comparison with theG(V)for KCNQ1/KCNE1 (thick black line). Thin lines show theG(V)(black) andF(V)(red) curves of KCNQ1 expressed alone for comparison.F1 andF2 represent the first and second fluorescence components (voltage sensor movements), respectively. The midpoints of activation for the fits are:G1/2=28.8±2.4 mV,F11/2=−97.4±7.05 mV,F21/2=23.0±7.2 mV; see Methods. (d) NormalizedG(V)s (black lines from a Boltzmann fit) andF(V)s (red or wine lines from a double Boltzmann fit) of recordings from KCNQ1/KCNE1 channels with positions 218, 219 and 221 (in S3–S4) mutated to cysteine (one at a time) and labelled with the fluorophores Alexa488-maleimide (red) or TMRM (wine). Data are mean±s.e.m.;n=4–7. (e) NormalizedF1(V)s andF2(V)s (solid and dashed lines from Boltzmann fit, respectively) fromd. Figure 1a shows the fluorescence (red) and current (black) measured simultaneously from KCNQ1/KCNE1 G219C channels in response to a family of voltage steps (−180 to +80 mV) from a prepulse to −140 mV. In response to the prepulse to −140 mV, the fluorescence signal decreases ( Fig. 1a , arrow), indicating that not all voltage sensors are in their resting position at the −80-mV holding potential. In response to depolarizing voltage pulses not activating ionic current (<−20 mV), the fluorescence change follows a monoexponential time course ( Fig. 1b , left). For voltage steps where channels open (≥−20 mV), two fluorescence components are present: one that is fast (purple dashed-dotted line) and develops well before the channel opens, and a second one that is slower (cyan dashed-dotted line) and develops with channel opening ( Fig. 1b , middle and right). Note that the fluorescence signals are much slower than the voltage changes, showing that the fluorescence changes are not because of direct effect of the voltage on the fluorophores per se . No fluorescence changes were detected from wild-type (wt) KCNQ1/KCNE1 channels treated with Alexa488-maleimide ( Supplementary Fig. 1a,b ), whereas qualitatively similar fluorescence changes, with a fast fluorescence change that develops before channel opening and an additional slow fluorescence change that develops with channel opening, were obtained from KCNQ1/KCNE1 channels with cysteine introduced at other positions in the S3–S4 loop and labelled with other fluorophores ( Supplementary Fig. 1c–j ). Figure 1: KCNE1 splits the voltage sensors movement of KCNQ1 into two components. ( a ) Representative current (black) and fluorescence (red) traces from KCNQ1/KCNE1 channels for the indicated voltage protocol (top). ( b ) Current (black) and fluorescence (red) in response to indicated test potentials for 5 s from −140 mV. The fluorescence traces are fit by a single exponential curve for the −80-mV step and a double exponential curve for the steps to −20 mV and +40 mV (black dashed line). The fast (purple dashed-dotted lines) and slow (cyan dashed-dotted lines) exponential curves of the double exponential fits are shown separately, overlaying the early and late part of the data, respectively. ( c ) Normalized G(V) (filled black circle and black line from a Boltzmann fit) and F(V) (open red circle and red line from a double Boltzmann fit) of recordings from KCNQ1/KCNE1 channels. The first (purple dashed-dotted lines) and the second (cyan dashed-dotted lines) Boltzmann curves of the double Boltzmann fits are shown separately, overlaying the data at negative and positive voltages, respectively. Data are mean±s.e.m. ; n =7. Cyan dashed line represents the second fluorescence component normalized between 0 and 1 for comparison with the G(V) for KCNQ1/KCNE1 (thick black line). Thin lines show the G(V) (black) and F(V) (red) curves of KCNQ1 expressed alone for comparison. F 1 and F 2 represent the first and second fluorescence components (voltage sensor movements), respectively. The midpoints of activation for the fits are: G 1/2 =28.8±2.4 mV, F 1 1/2 =−97.4±7.05 mV, F 2 1/2 =23.0±7.2 mV; see Methods. ( d ) Normalized G(V) s (black lines from a Boltzmann fit) and F(V) s (red or wine lines from a double Boltzmann fit) of recordings from KCNQ1/KCNE1 channels with positions 218, 219 and 221 (in S3–S4) mutated to cysteine (one at a time) and labelled with the fluorophores Alexa488-maleimide (red) or TMRM (wine). Data are mean±s.e.m. ; n =4–7. ( e ) Normalized F 1 (V) s and F2(V) s (solid and dashed lines from Boltzmann fit, respectively) from d . Full size image The dissociation of the fluorescence from KCNQ1/KCNE1 channels into two kinetic components is paralleled in the steady-state fluorescence versus voltage curve, F(V) , which is also split into two components ( Fig. 1c , open red circle). The F(V) ( Fig. 1c ) is fit by the sum of two Boltzmann distributions (red thick line): one at negative voltages (purple dashed-dotted line) and another one at positive voltages (cyan dashed-dotted line). Notably, the normalized second F(V) component (dashed cyan line) fairly well follows the steady-state conductance versus voltage curve, G(V) ( Fig. 1c , filled black circle). In contrast to KCNQ1/KCNE1 channels, the F(V) curve from KCNQ1 alone is well fit by a single Boltzmann distribution that overlays well with the G(V) of KCNQ1 channels ( Fig. 1c , red and black thin lines [13] ). The F(V) s from KCNQ1/KCNE1 channels with other positions in S3–S4 mutated to cysteines and other fluorophores also displayed two Boltzmann distributions: one at negative voltages and one at more positive voltages ( Fig. 1d ), similar to Alexa488-labelled 219C KCNQ1/KCNE1 channels ( Fig. 1e ). The results in Fig. 1 show that the fluorescence from a fluorophore in the S3–S4 loop in KCNQ1/KCNE1 channels is clearly divided into two components that we will call F 1 and F 2, and that F 2 correlates with channel opening. S4 accessibility supports two components of S4 movement To assess the relation between S4 movement and the two fluorescence components F 1 and F 2, we use the rate of access for externally applied membrane-impermeable cysteine reagent 2-(Trimethylammonium)ethyl]methanethiosulfonate Bromide (MTSET) to cysteines introduced in S4 as an independent assay. We individually mutated residues A223 and T224 to cysteine in the S4 domain. Perfusion of external MTSET modifies KCNQ1/KCNE1 A223C channels at 0 mV ( Fig. 2a ), the voltage where the first component of the fluorescence F 1 is near saturation ( Fig. 1c ). The MTSET modification accelerates the activation of KCNQ1/KCNE1 A223C channels ( Fig. 2a ). External MTSET modified A223C 10-fold faster at 0 mV than at −80 mV ( Fig. 2b ). The modification rates for 223C and 224C approach zero at −140 mV, as if both residues become inaccessible from the extracellular solution ( Fig. 2c ). When KCNQ1 is coexpressed with KCNE1, residue 223 is accessible to MTSET at 0 mV, whereas residue 224 requires positive voltages to become accessible with a comparable rate ( Fig. 2c ). Although the voltage dependence of the modification rate of A223C (black circle) follows the voltage dependence of the first fluorescence component F 1, the voltage dependence of T224C (purple triangle) follows the voltage dependence of the second fluorescence component F 2, suggesting that S4 moves in two steps ( Fig. 2c ). In contrast, in the absence of KCNE1, the cysteine modification rates of 223C and 224C in KCNQ1 follow the voltage dependence of the monophasic fluorescence in KCNQ1 alone ( Fig. 2e ). These results suggest that S4 moves in one step (or two steps with overlapping voltage dependences) in KCNQ1 channel alone ( Fig. 2f ) and in two steps (that correlates with fluorescence components F 1 and F 2) with widely different voltage dependences in KCNQ1/KCNE1 channels ( Fig. 2e ). These accessibility data further suggest that S4 undergoes conformational changes during both fluorescence components. However, it is also possible that the second fluorescence change reports on conformational changes in the pore domain during opening that indirectly affects the environment of the fluorophore. 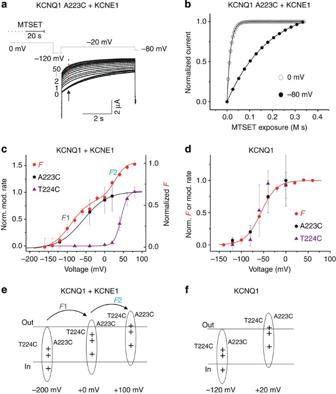Figure 2: S4 residue accessibility shows two components of S4 movement in KCNQ1/KCNE1 channels. (a) Current in response to a −20 mV voltage step before (trace 0) and during (traces 1–50) membrane-impermeable thiol reagent MTSET application on KCNQ1/KCNE1 A223C channels. External MTSET is applied at 0 mV for 20 s and then washed away for 12 s, before the cell is hyperpolarized to −120 mV for 12 s, as indicated by the voltage protocol (seeSupplementary Fig. 2for details). (b) MTSET modification rates at 0 and −80 mV using the current amplitudes measured at the arrow ina. (c,d) Normalized (Norm.) voltage dependence of the modification (Mod.) rate for MTSET to residues 223C (black circle) and 224C (purple triangle) in (c) KCNQ1/KCNE1 and (d) KCNQ1 channels. Data are mean±s.e.m. for 5–8 cells in each group. NormalizedF(V)(red) is shown for comparison. (e,f) Cartoon models depicting voltage sensor movement in two steps in (e) KCNQ1/KCNE1 channels and in one step (f) KCNQ1 channel alone, respectively. Figure 2: S4 residue accessibility shows two components of S4 movement in KCNQ1/KCNE1 channels. ( a ) Current in response to a −20 mV voltage step before (trace 0) and during (traces 1–50) membrane-impermeable thiol reagent MTSET application on KCNQ1/KCNE1 A223C channels. External MTSET is applied at 0 mV for 20 s and then washed away for 12 s, before the cell is hyperpolarized to −120 mV for 12 s, as indicated by the voltage protocol (see Supplementary Fig. 2 for details). ( b ) MTSET modification rates at 0 and −80 mV using the current amplitudes measured at the arrow in a . ( c , d ) Normalized (Norm.) voltage dependence of the modification (Mod.) rate for MTSET to residues 223C (black circle) and 224C (purple triangle) in ( c ) KCNQ1/KCNE1 and ( d ) KCNQ1 channels. Data are mean±s.e.m. for 5–8 cells in each group. Normalized F(V) (red) is shown for comparison. ( e , f ) Cartoon models depicting voltage sensor movement in two steps in ( e ) KCNQ1/KCNE1 channels and in one step ( f ) KCNQ1 channel alone, respectively. Full size image Gating currents in KCNQ1/KCNE1 channels To test how the fluorescence signal relates to the S4 charge movements, we measure ON gating currents ( I gON ) using the cut-open voltage clamp technique on oocytes expressing KCNQ1/KCNE1 channels in the absence of permeant K + ions (see Methods). If the fluorescence probe reports on S4 charge movement, a charge movement in KCNQ1/KCNE1 channel is expected to occur in the voltage range from −180 to +100 mV ( Fig. 1c ). To detect such charge movements, cells expressing KCNQ1/KCNE1 channels are held at −140 mV and depolarized to test potentials ranging from −40 to +80 mV ( Fig. 3a ). In response to this protocol much of the fluorescence change is fast ( Fig. 1a ), so that an associated gating current might be detectable (for a given charge movement, the amplitude of gating current is inversely related to the time constant). Indeed, we detect charge movements in KCNQ1/KCNE1 channels in response to depolarization ( Fig. 3a ). Charge movements following repolarization to −140 mV are not resolved, as expected from the slow-off kinetics of fluorescence and K + current. The first fluorescence component F 1 and the integrated gating charge ( Q ON =integral of I gON ) have similar kinetics at voltages >−20 mV ( Fig. 3b ). At more negative voltages, gating currents are not reliably detected. The slow kinetics of the fluorescence at these negative voltages suggests that gating currents are too slow (and thereby too small) to be detected in this voltage range. Therefore, we measure the voltage dependence of the gating charge movement, Q(V), by a prepulse protocol in which we first pre-equilibrate the channels by stepping to voltages between −180 and +100 mV for 5 s, then measure the gating currents in response to a fixed voltage step to +80 mV ( Fig. 3c ). The Q(V) curve measured by this protocol overlaps the first fluorescence component F 1 of the F(V) curve ( Fig. 3d ), as if F 1 is approximately proportional to the main gating charge moved in KCNQ1/KCNE1 channels. Some gating charge must move in the conformational change underlying the second fluorescence component F 2, but likely moves too slowly to be reliably measured. That the kinetics and voltage dependence of the gating currents from wt KCNQ1/KCNE1 channels closely resemble the fluorescence component F 1 further supports that the fluorescence at negative voltages in Alexa488-labelled 219C KCNQ1/KCNE1 channels reliably report on S4 charge movement. 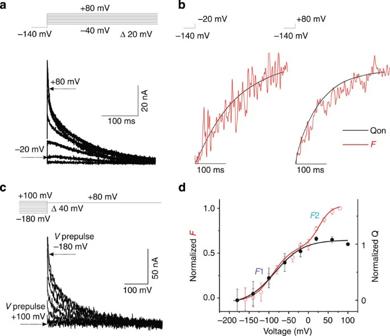Figure 3: Gating currents in KCNQ1/KCNE1 channels follow the first fluorescence component. (a) Representative gating current from KCNQ1/KCNE1 channels using the voltage protocol indicated (top). (b) Normalized fluorescence (red) and the integrated gating charge (black) QONin response to −20 and +80 mV pulses for 300 ms. (c) Representative gating current from KCNQ1/KCNE1 channels using a prepulse protocol by stepping to voltages between −180 and +100 mV for 5 s, before measuring the gating currents in response to a fixed voltage step to +80 mV. Each prepulse moves different amount of gating charge (0 toQmaxaccording to theQ(V)) and the remaining gating chargeQmeasured(=Qmax−Q(V) ) is moved during the following pulse to +80 mV. (d) NormalizedQ(V)(solid black circle and black line from a Boltzmann fit) measured from experiments as inc. Data are mean±s.e.m.;n=3. TheQ(V)was calculate from the integrated gating currents,Qmeasured(V), incduring the +80 mV step asQ(V)=Qmax−Qmeasured(V). NormalizedF(V)as inFig. 1c(open red circle and red line from a double Boltzmann fit) is shown for comparison.Q1/2=−84.2±9.8 mV; seeFig. 1cforF11/2andF21/2, respectively. Note thatQ(V)overlaps the first fluorescence componentF1 of theF(V)in KCNQ1/KCNE1 channels. Figure 3: Gating currents in KCNQ1/KCNE1 channels follow the first fluorescence component. ( a ) Representative gating current from KCNQ1/KCNE1 channels using the voltage protocol indicated (top). ( b ) Normalized fluorescence (red) and the integrated gating charge (black) Q ON in response to −20 and +80 mV pulses for 300 ms. ( c ) Representative gating current from KCNQ1/KCNE1 channels using a prepulse protocol by stepping to voltages between −180 and +100 mV for 5 s, before measuring the gating currents in response to a fixed voltage step to +80 mV. Each prepulse moves different amount of gating charge (0 to Q max according to the Q(V) ) and the remaining gating charge Q measured ( =Q max −Q(V ) ) is moved during the following pulse to +80 mV. ( d ) Normalized Q(V) (solid black circle and black line from a Boltzmann fit) measured from experiments as in c . Data are mean±s.e.m. ; n =3. The Q(V) was calculate from the integrated gating currents, Q measured (V) , in c during the +80 mV step as Q(V)=Q max −Q measured (V) . Normalized F(V) as in Fig. 1c (open red circle and red line from a double Boltzmann fit) is shown for comparison. Q 1/2 =−84.2±9.8 mV; see Fig. 1c for F 1 1/ 2 and F 2 1/ 2 , respectively. Note that Q(V) overlaps the first fluorescence component F 1 of the F(V) in KCNQ1/KCNE1 channels. Full size image First component of fluorescence isolated pharmacologically As we detect two fluorescence changes, one at negative potentials ( F 1) that has a similar kinetics as the gating current and another at positive potentials ( F 2) that correlates with channel opening, we hypothesize that F 1 reports on the main S4 gating charge movement and F 2 reports on a late conformational change of S4 during channel opening ( Fig. 4f upper cartoon). We reason that if the second conformational change of S4 is coupled to channel opening, then locking the S6 gate in a closed state by a suitable blocker would impede the late S4 motion. 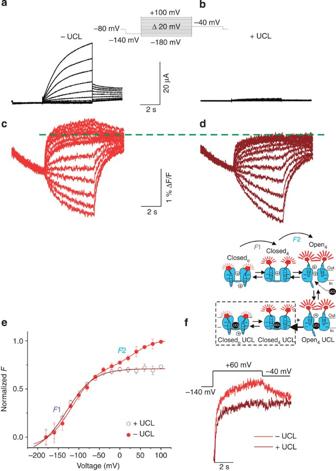Figure 4: UCL 2077 isolated the first component of the fluorescence change. Representative current (a,b) and fluorescence (c,d) traces from KCNQ1/KCNE1 channels before (a,c) and during (b,d) extracellular application of UCL 2077 (UCL 2077 is lipid permeable). Cells are held at −80 mV and prepulsed to −140 mV for 3 s before stepping to potentials between −180 and +100 mV in 20-mV intervals for 5 s, followed by pulse to −40 mV for 5 s to record tail currents. Green dashed line is shown to denote the absence of the second fluorescence component during application of UCL 2077. (e) NormalizedF(V)of recordings from KCNQ1/KCNE1 channels before (filled red circle) and during (open wine red circle) application of UCL 2077. Data are mean±s.e.m.;n=5. (f) Time course of fluorescence in response to a +60-mV pulse for 5 s before (red) and during (wine red) application of UCL 2077. (Inset) Cartoon consistent with the effect of UCL 2077 on KCNQ1/KCNE1 channel gating. Once the channel opens, the open-channel blocker UCL 2077 ref.20access its binding site in the pore. UCL 2077 promotes gate closing by binding to the S6 gate. The first fluorescence component is not affected by UCL 2077 binding (dashed square), but the second S4 movement and channel opening are inhibited. Figure 4: UCL 2077 isolated the first component of the fluorescence change. Representative current ( a , b ) and fluorescence ( c , d ) traces from KCNQ1/KCNE1 channels before ( a , c ) and during ( b , d ) extracellular application of UCL 2077 (UCL 2077 is lipid permeable). Cells are held at −80 mV and prepulsed to −140 mV for 3 s before stepping to potentials between −180 and +100 mV in 20-mV intervals for 5 s, followed by pulse to −40 mV for 5 s to record tail currents. Green dashed line is shown to denote the absence of the second fluorescence component during application of UCL 2077. ( e ) Normalized F(V) of recordings from KCNQ1/KCNE1 channels before (filled red circle) and during (open wine red circle) application of UCL 2077. Data are mean±s.e.m. ; n =5. ( f ) Time course of fluorescence in response to a +60-mV pulse for 5 s before (red) and during (wine red) application of UCL 2077. (Inset) Cartoon consistent with the effect of UCL 2077 on KCNQ1/KCNE1 channel gating. Once the channel opens, the open-channel blocker UCL 2077 ref. 20 access its binding site in the pore. UCL 2077 promotes gate closing by binding to the S6 gate. The first fluorescence component is not affected by UCL 2077 binding (dashed square), but the second S4 movement and channel opening are inhibited. Full size image To test this hypothesis, we measure fluorescence changes before and during application of UCL 2077, an open-channel blocker of KCNQ1 channels [20] . Bath perfusion of 10 μM UCL 2077 inhibits ionic current of KCNQ1/KCNE1 channels almost completely ( Fig. 4a,b ). In contrast, 10 μM of UCL 2077 does not abolish the fluorescence change ( Fig. 4c,d ). However, UCL 2077 eliminates the second component of the fluorescence change observed at positive potentials ( Fig. 4d,e , filled red circle versus wine red open circle). Figure 4f superimposes the time courses of fluorescence change for KCNQ1/KCNE1 recorded before and during application of UCL 2077. UCL 2077 eliminates the second, slow fluorescence component, so that the time course of fluorescence change in the presence of UCL 2077 is fast and monoexponential ( Fig. 4f , wine red line). The fluorescence change is reduced to that described as F 1 in Fig. 1b,c and reflected in the integrated gating current ( Fig. 3b,d ). These data suggest that the second fluorescence change eliminated by UCL 2077 appears to report on an additional S4 movement that is associated with channel opening. The effect of UCL 2077 on KCNQ1/KCNE1 channels is similar to the effect of 4-AP on Shaker K + channels [21] . 4-aminopyridine (4-AP) is thought to block open Shaker K + channels and then to stabilize S6 (the gate) in the closed position, thus preventing the gate from re-opening [21] . In analogy to 4-AP’s effect on Shaker K + channels, we propose that UCL 2077 binds to S6 in the pore when KCNQ1/KCNE1 channels open. Once UCL 2077 has bound to the pore, it stabilizes the gate in the closed state, thereby preventing reopening of the gate and the second S4 movement (cartoon in Fig. 4f ). In contrast to UCL 2077, the KCNQ1/KCNE1 channel blocker chromanol 293B has only minor effect on the voltage sensor movement ( Supplementary Fig. 3 ), most likely because it binds to the selectivity filter of KCNQ1 channel [22] and not to the S6 gate. Fluorescence components are further separated by a mutation A mutation in KCNE1, K70N, causes long-QT-syndrome [23] . The G(V) relation of KCNQ1/KCNE1 K70N channels is right-shifted compared with wt KCNQ1/KCNE1 channels [24] . We reason that if the second fluorescence component F 2 reports on a conformational change of S4 associated with channel opening, then in KCNQ1/KCNE1 K70N channels F 2 should be equally shifted to more positive potentials. 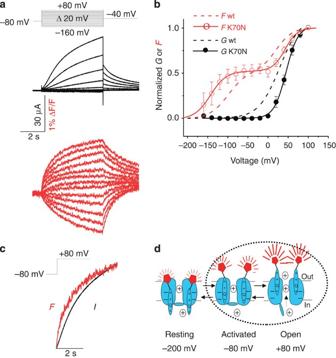Figure 5: K70N in KNCE1 farther separates the two voltage sensor movements of KCNQ1. (a) Representative current (black) and fluorescence (red) traces from KCNQ1 channel coexpressed with KCNE1 K70N mutant in response to the indicated protocol (top). (b) NormalizedG(V)(filled black circle and black line from a Boltzmann fit) andF(V)(open red circle and red line from a double Boltzmann fit) of recordings from KCNQ1/KCNE1 K70N channels. Data are mean±s.e.m.;n=7. Dashed lines represent wt KCNQ1/KCNE1G(V)(black) andF(V)(red) curves for comparison. K70NG1/2=44.8±0.9, K70NF11/2=−143.0±13.0 mV, K70NF21/2=42.3±2.6 mV; seeFig. 1cfor wtF11/2andF21/2. (c) Time course of current (black) and fluorescence (red) in response to +80 mV pulse for 5 s. (d) Cartoon of KCNQ1/KCNE1 K70N gating. At −80 mV, K70N channels are mainly in the activated closed state, so a depolarization from −80 mV will only show mainly the slow fluorescence component that correlates with channel opening. Figure 5a shows the current (black) and fluorescence (red) from KCNQ1/KCNE1 K70N channels. The KCNE1 K70N mutation further separates the two components apparent in the F(V) relation ( Fig. 5b , open red circle). The first component F 1 in the F(V) is left-shifted in K70N compared with wt (dashed red line), whereas F 2 is right-shifted and follows the G(V) (filled black circle) that is also right-shifted in K70N compared with wt (dashed black line, Fig. 5b ). The time course of the fluorescence change during a depolarization to +80 mV from −80 mV (where most of F 1 is completed), closely follows the time course of channel opening ( Fig. 5c ), as if F 2 and channel opening are because of the same concerted conformational change ( Fig. 5d ). Figure 5: K70N in KNCE1 farther separates the two voltage sensor movements of KCNQ1. ( a ) Representative current (black) and fluorescence (red) traces from KCNQ1 channel coexpressed with KCNE1 K70N mutant in response to the indicated protocol (top). ( b ) Normalized G(V) (filled black circle and black line from a Boltzmann fit) and F(V) (open red circle and red line from a double Boltzmann fit) of recordings from KCNQ1/KCNE1 K70N channels. Data are mean±s.e.m. ; n =7. Dashed lines represent wt KCNQ1/KCNE1 G(V) (black) and F(V) (red) curves for comparison. K70N G 1/2 =44.8±0.9, K70N F 1 1/2 =−143.0±13.0 mV, K70N F 2 1/2 =42.3±2.6 mV; see Fig. 1c for wt F 1 1/2 and F 2 1/2 . ( c ) Time course of current (black) and fluorescence (red) in response to +80 mV pulse for 5 s. ( d ) Cartoon of KCNQ1/KCNE1 K70N gating. At −80 mV, K70N channels are mainly in the activated closed state, so a depolarization from −80 mV will only show mainly the slow fluorescence component that correlates with channel opening. Full size image Isolating phases of gating by VCF protocols Our data suggests that KCNQ1/KCNE1 channel gating occurs in two phases that we call F 1 and F 2. Upon depolarization, a first step (with rate α) involves S4s movement from a resting to an activated state without opening the conducting pore. This is then followed by a second rearrangement of S4 (with rate γ) upon channel opening ( Fig. 5d ). Upon hyperpolarization, channels close in the reverse order. S4 first rearranges back to its activated position during channel closing (with rate δ), then it moves back to its resting state (with rate β) ( Fig. 5d ). To determine the rates and voltage dependence of the different transitions, we design four different protocols to measure the transitions separately ( Fig. 6a,c,e,g ). First, to estimate the rate α, we determine the time constant τ α of the fast fluorescence component in response to different activation voltage steps ( Fig. 6a,b ). τ α approximates 1/α for large depolarizations. The effective gating charge calculated from the voltage dependence of α is z α =0.39±0.021 e 0 , ( n =5) ( Fig. 6b ). 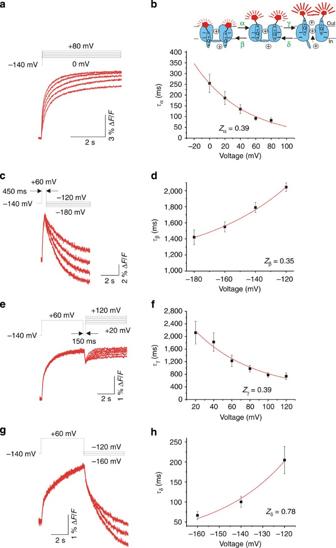Figure 6: Isolating rate constants in KCNQ1/KCNE1 channels by VCF protocols. (a,c,e,g) Representative fluorescence traces in response to four different voltage protocols (top) to estimate: (a) rate-α, (c) rate-β, (e) rate-γ and (g) rate-δ. (b,d,f,h) Voltage dependence of the time constantτ(which approximate (b) 1/α, (d) 1/β, (f) 1/γ and (h) 1/δ) from data recorded as ina,c,e,g, respectively,.τβandτγ, were determined by fitting traces as shown incandewith a single exponential.τα, andτδwere determined by fitting traces as shown inaandgwith a double exponential and using the fast time constant. Data inb,d,f,hwere fitted withτ(V)=τ(0)/exp(−zFV/RT). Data inb,d,f,hare mean±s.e.m.;n=4–6. (Inset) Cartoon representing a model of KCNQ1/KCNE1 channel gating with the respective rate constants. Figure 6: Isolating rate constants in KCNQ1/KCNE1 channels by VCF protocols. ( a , c , e , g ) Representative fluorescence traces in response to four different voltage protocols (top) to estimate: ( a ) rate-α, ( c ) rate-β, ( e ) rate-γ and ( g ) rate-δ. ( b , d , f , h ) Voltage dependence of the time constant τ (which approximate ( b ) 1/α, ( d ) 1/β, ( f ) 1/γ and ( h ) 1/δ) from data recorded as in a , c , e , g , respectively,. τ β and τ γ , were determined by fitting traces as shown in c and e with a single exponential. τ α , and τ δ were determined by fitting traces as shown in a and g with a double exponential and using the fast time constant. Data in b , d , f , h were fitted with τ(V)=τ(0)/ exp(− zFV/RT) . Data in b , d , f , h are mean±s.e.m. ; n =4–6. (Inset) Cartoon representing a model of KCNQ1/KCNE1 channel gating with the respective rate constants. Full size image To isolate β ( Fig. 6c ), we first apply a step to +60 mV for 450 ms to allow the channel to undergo α without much γ (that is, no channel opening). Subsequently, we step down to different negative voltages for 5 s to allow the channel to undergo β and measured τ β ( Fig. 6d ). τ β approximates 1/β for large hyperpolarizations. The calculated effective gating charges for β is z β =0.35±0.09 e 0 , ( n =5) ( Fig. 6d ). Next, we isolate γ from α by first opening the channel at +60 mV for 5 s. Following channel opening, a 150-ms pulse to −140 mV allows the channel to undergo δ without much β. Reopening to different positive voltages, let us measure τ γ (approximately 1/γ) ( Fig. 6e,f ). During this second depolarizing pulse, the channel only goes through γ, because the channels have already undergone α during the first depolarizing pulse (cartoon in Fig. 6 ). τ γ approximates 1/γ for large depolarizations. The effective gating charge calculated for the voltage dependence of γ is z γ =0.39±0.082 e 0 , ( n =4) ( Fig. 6f ). The rate δ is measured by opening the channel for 5 s at +60 mV, followed by stepping to different negative voltages for 5 s ( Fig. 6g ). In response to the hyperpolarizing pulses, the fluorescence decays with two components ( Fig. 6g ). The fast fluorescence component is interpreted as the channel undergoing δ, because β takes place at much slower rate (compare Fig. 6c,g ). τ δ approximates 1/δ for large hyperpolarizations. The calculated effective gating charges for δ is z δ =0.78±0.07 e 0 , ( n =4) ( Fig. 6h ). Model for KCNQ1/KCNE1 channel gating We use the estimates of the different rate constants and their voltage dependences from Fig. 6 to construct the six-state scheme for KCNQ1/KCNE1 channels in Fig. 7a . In the six-state model, we assume that the main gating charge movement of the four voltage sensors occurs independently in the four subunits, and that a concerted further movement of gating charge in all four subunits occurs during channel opening ( Fig. 7a ). Because we observe a fluorescence component that is associated with channel opening, we assume that all four S4s move and thereby generate a fluorescence component during the opening step ( Fig. 7a ). We assume that this second S4 conformational change is concerted in all four subunits, because the fluorescence and ionic currents follow each other in the K70N mutant ( Fig. 5c ). KCNQ1/KCNE1 channels have been shown to have several subconductance states [25] . However, the transitions between different subconductance levels are relatively fast compared with the first opening and the first latency to the smallest subconductance level that correlates with channel opening [25] . Therefore, we restrict our model to only one open conductance level. In this model, the measured z α + z β =0.74 e 0 is the charge moved in each subunit during F 1, whereas z γ + z δ =1.17 e 0 is the total charge moved during F 2. Therefore, the total gating charge for KCNQ1/KCNE1 channels according to this model is 4.13 e 0 /channel (= 4 × ( z α + z β )+( z γ + z δ )). This model can well reproduce the current and fluorescence of KCNQ1/KCNE1 channels ( Fig. 7b–d ; note that all parameters are set by the experiments in Fig. 6 ). Differences between our six-state model and experimental data are expected because our protocols in Fig. 6 do not fully isolate the different rate constants. The model in Fig. 7a reproduces the KCNQ1/KCNE1 biophysical characteristics (compared with KCNQ1 expressed alone [26] ): the main voltage sensor movement is shifted to more negative potentials, the opening of the gate is shifted to more positive potentials, and the kinetics of opening is slowed ( Fig. 7c,d ). In response to depolarizations from a holding voltage of −140 mV, our KCNQ1/KCNE1 model displays an early fast fluorescence component, as each voltage sensor moves from a resting position to an activated position (channel states C 0 –C 4 in Fig. 7a ). A late slow fluorescence component follows at depolarizations to positive voltages ( Fig. 7b,c ), when all four voltage sensors undergo an additional, concerted conformation change that opens the channel (C 4 –O 4 in Fig. 7a ). The time it takes to transitions from the resting position to C 4 accounts for the delay ( Fig. 7d ) in the sigmoidal activation time course of the ionic currents in KCNQ1/KCNE1 channels. The model also reproduces fairly well the experimental gating current of KCNQ1/KCNE1 ( Fig. 7e ), with differences at voltages >+60 mV, for which the experimental charge movement is slightly faster than predicted by the model. To fit the details of the complex kinetics of the gating currents (slight rise phase at lower voltages and bi-exponential at more depolarized voltages; Fig. 3a ) a more complex model would be necessary. By setting the transition rate between C 4 and O 4 to 0 to prevent channel opening, the model also reproduces the effect of UCL on the fluorescence ( Fig. 7f ). By slowing slow down the return of the main voltage sensor movement (β) and the opening conformational change (γ), our model reproduces fairly well the results from K70N ( Fig. 7g,h ). 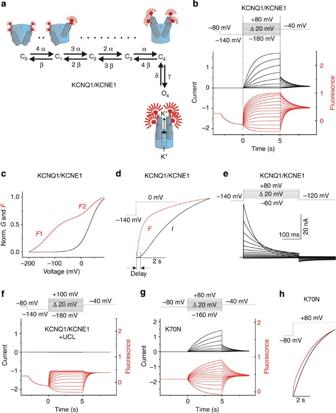Figure 7: Model for KCNQ1/KCNE1 channel gating. (a) A six-state allosteric gating scheme for KCNQ1/KCNE1 channels. Horizontal transitions represent independent S4 movements that increase the fluorescence to an intermediate level. The vertical transition represents concerted channel opening with a concomitant additional fluorescence increase. Cartoon shows KCNQ1 channel labelled with a fluorophore on S3–S4 with all four voltage sensors in the resting state (C0), with one (C1), or four (C4) voltage sensor activated without channel opening (top) that is followed by a concerted conformational change of all four S4s associated with channel opening (O4; bottom). (b) Model simulation of current (black) and fluorescence (red) for KCNQ1/KCNE1 channel using the indicated voltage protocol (top). Note that all parameters in the model are determined by the estimates of the different rate constants and their voltage dependences fromFig. 6(Supplementary Table 1). Current and fluorescence traces were simulated using Berkeley Madonna (Berkeley, CA, USA). (c) SimulatedG(V)andF(V)curves for KCNQ1/KCNE1 channels from simulation inb. Norm., normalized. (d) Model simulation for activation time course of current (black) and fluorescence (red) at 0 mV (fromb) in KCNQ1/KCNE1 channels. (e) Model simulation of gating currents in KCNQ1/KCNE1 channels using the indicated voltage protocol (top) and same parameters as inb. (f) Model simulation of current (black) and fluorescence (red) for KCNQ1/KCNE1 channel in the presence of UCL 2077 using the indicated voltage protocol (top). Same parameters as inb, except thatγ=0 to prevent channel opening. (g) Model simulation of current (black) and fluorescence (red) from KCNQ1/KCNE1 K70N channels using the indicated voltage protocol (top). Same parameters as inb, except thatβandδare slowed down compared with wt to shiftF1 by −40 mV andF2 by +20 mV as inFig. 5b. (h) Model simulation for activation time course of current (black) and fluorescence (red) at +80 mV (fromg) in KCNQ1/KCNE1 K70N channels. Figure 7: Model for KCNQ1/KCNE1 channel gating. ( a ) A six-state allosteric gating scheme for KCNQ1/KCNE1 channels. Horizontal transitions represent independent S4 movements that increase the fluorescence to an intermediate level. The vertical transition represents concerted channel opening with a concomitant additional fluorescence increase. Cartoon shows KCNQ1 channel labelled with a fluorophore on S3–S4 with all four voltage sensors in the resting state (C 0 ), with one (C 1 ), or four (C 4 ) voltage sensor activated without channel opening (top) that is followed by a concerted conformational change of all four S4s associated with channel opening (O 4 ; bottom). ( b ) Model simulation of current (black) and fluorescence (red) for KCNQ1/KCNE1 channel using the indicated voltage protocol (top). Note that all parameters in the model are determined by the estimates of the different rate constants and their voltage dependences from Fig. 6 ( Supplementary Table 1 ). Current and fluorescence traces were simulated using Berkeley Madonna (Berkeley, CA, USA). ( c ) Simulated G(V) and F(V) curves for KCNQ1/KCNE1 channels from simulation in b . Norm., normalized. ( d ) Model simulation for activation time course of current (black) and fluorescence (red) at 0 mV (from b ) in KCNQ1/KCNE1 channels. ( e ) Model simulation of gating currents in KCNQ1/KCNE1 channels using the indicated voltage protocol (top) and same parameters as in b . ( f ) Model simulation of current (black) and fluorescence (red) for KCNQ1/KCNE1 channel in the presence of UCL 2077 using the indicated voltage protocol (top). Same parameters as in b , except that γ =0 to prevent channel opening. ( g ) Model simulation of current (black) and fluorescence (red) from KCNQ1/KCNE1 K70N channels using the indicated voltage protocol (top). Same parameters as in b , except that β and δ are slowed down compared with wt to shift F 1 by −40 mV and F 2 by +20 mV as in Fig. 5b . ( h ) Model simulation for activation time course of current (black) and fluorescence (red) at +80 mV (from g ) in KCNQ1/KCNE1 K70N channels. Full size image The mechanism of how KCNE1 interacts with KCNQ1 to alter the channel properties is currently a matter of intense debate. Is the activation of KCNQ1/KCNE1 channels slow because KCNE1 slows the movement of the voltage sensors, or because KCNE1 slows the opening of the gate, or a combination of both? Our results, based on VCF and cysteine accessibility, show that KCNE1 separates the voltage sensor (S4) movement of KCNQ1 channel into two components: a rapid S4 movement occurs at negative voltages well before channel opening and a slow S4 movement that occurs at positive voltages and parallels channel opening. The two components can be pharmacologically separated by the KCNQ1 blocker UCL 2077 and further separated by the Long QT mutation K70N in KCNE1. Gating currents develop with a similar time and voltage dependence as the first fluorescence component F 1, as if F 1 reports on the main S4 charge movement. The voltage dependence of F 1 correlates with the voltage range of Cole–Moore shifts [13] , as if the first component of S4 movement is necessary for channel opening. Using a six-state model with all rates determined from our experiments ( Fig. 6 ), we can reproduce all of our results on KCNQ1/KCNE1 channels ( Fig. 7 ). In this model, KCNQ1/KCNE1 channel has a fast S4 movement at negative voltages that moves the majority of gating charge and a slower second conformational change at positive voltages that moves a smaller amount of gating charge and opens the gate. Other models, with a slow S4 movement and a fast gate opening, have been proposed to explain the characteristics of KCNQ1/KCNE1 channels [25] , [27] , [28] ( Supplementary Fig. 4f ). In contrast to our model ( Fig. 7a ), these models cannot reproduce the current and fluorescence from a triple pulse protocol ( Supplementary Fig. 4 ) or from the protocols shown in Fig. 6c or e . However, a recent study concluded that KCNE1 slows the movement of the voltage sensor movement, and that the voltage sensor movement is the rate-limiting step for channel opening in KCNQ1/KCNE1 channels [12] , because the authors could not measure gating current from KCNQ1 channels in the presence of KCNE1 and, for depolarization from a holding potential of −90 mV, the kinetics and voltage dependence of the ionic current and the fluorescence were similar. In contrast, we find that if we hold the channels at large negative voltages and step to positive voltages, the majority of the fluorescence occurs much faster than the current ( Supplementary Fig. 5 ). The fact that Ruscic et al. used Tetramethylrhodamine-5-maleimide (TMRM) as their fluorescence reporter [12] , which displays a smaller first fluorescence component ( Fig. 1d ) than the fluorophore we mainly used (Alexa488-maleimide), could explain partly why they missed the first fluorescence component. We find that the difference between the kinetics of S4 movement and channel opening is decreased if stepped from less-negative voltages ( Supplementary Fig. 5 ). We interpret these results as follows: during depolarization from very negative holding voltages all four S4s move from the resting state to the activated state, thereby generating the fast fluorescence signal in a time frame that correlates with the initial delay of the current; then a slower conformational change of S4 is coupled to the time course of channel opening ( Fig. 7 ). In contrast, if the depolarization starts from less-negative holding voltages ( Supplementary Fig. 5 ), or if the first S4 charge movement occurs at very negative voltages as in the K70N mutation ( Fig. 5 ), then some, or all, of the channels are already in the activated state (C 4 ). Therefore, the fast fluorescence signal will be small, or absent, and instead the majority of the fluorescence signal will correlate with the slower time course of channel opening. Thus, in addition to differences in fluorophores used, differences in voltage protocols might explain part of the differences between our and Ruscic et al. [12] results. The fact that Ruscic et al. [12] looked for gating currents in the voltage range where our results suggest that most S4s are already activated may explain why they could not measure gating current from KCNQ1/KCNE1 channels. In contrast, by holding at more negative voltages, we were able to measure gating currents that correlated with the fast fluorescence component F 1 ( Fig. 3 ). It is important to note that at the diastolic potential in a ventricular myocyte (−90 mV), approximately half of the voltage sensors will be in the resting state ( Fig. 1c ). In our model, the movement of these voltage sensors from the resting to the activated position during the systolic depolarization generates the physiologically important initial delay in the I Ks (KCNQ1/KCNE1) currents. Our experiments suggests that the total gating charge for a KCNQ1/KCNE1 channel is 4.13 e 0 , substantially lower than for Shaker K channels (12–13 e 0 ) (refs 29 , 30 , 31 ). However, there are only three arginines in S4 of KCNQ1, compared with seven positively charged amino acids in S4 of Shaker. The homologous residues in Shaker to two of the missing arginines (R3 and R5) have been shown to contribute 1 and 0.5 charges per subunit, respectively [31] , suggesting that S4 in KCNQ1/KCNE1 channels undergo a similar, or slightly smaller, transmembrane movement than Shaker, but with fewer charged S4 residues. Comparing our models developed using VCF for KCNQ1 expressed alone [26] and for KCNQ1 coexpressed with KCNE1 allows us to understand how KCNE1 affects KCNQ1 channels: KCNE1 stabilizes the activated closed state (state C 4 ; Fig. 7a ). This causes the S4 movement to split into two steps: the main voltage sensor movement is shifted to more negative voltages, whereas the second S4 movement and channel opening are shifted to more positive voltages and slowed down. In addition, KCNE1 destabilizes the open states with <4 activated S4s, so that, in contrast to KCNQ1 alone [26] , KCNQ1/KCNE1 channels do not open until all four S4s have activated [13] , [26] . This model for KCNQ1/KCNE1 channels, in combination with VCF data, also allows us to better understand the molecular mechanism underlying disease-causing mutations in KCNQ1/KCNE1. For example, we show that the KCNE1 K70N mutation shifts the F 1 and F 2 fluorescence components in opposite directions along the voltage axis. We interpret this as if the K70N mutation further stabilizes the closed activated state C 4 (with all four S4s activated), thereby shifting the main voltage sensor movement ( F 1) to negative voltages while shifting channel opening (and F 2) to more positive voltages compared with wt KCNQ1/KCNE1 channels. Importantly, understanding the effect of a disease-causing mutation on the voltage sensor movement and the gate can lead to a better understanding of the molecular mechanism underlying the defect caused by the mutation, which can lay the groundwork for developing future therapeutic agents to treat these diseases. In summary, our study demonstrates that KCNE1 alters the kinetics and voltage dependence of voltage sensor activation and channel opening of KCNQ1 channels. The characteristic activation delay in KCNQ1/KCNE1 channels is explained by a relatively fast (compared with the ionic current kinetics) main charge movement. The slow kinetics of KCNQ1/KCNE1 channels following the initial delay is because of a second, slower conformational change that further moves S4 and opens the channel. Our results show that the voltage dependence of the main gating charge movement and channel opening are separated by >100 mV in KCNQ1/KCNE1 channels. This is very different from other voltage-gated cation channels, for which the gating charge movement and channel opening are tightly coupled [32] , [33] . Molecular biology We used human KCNQ1 and KCNE1 subcloned into the pGEM-HE oocyte expression vector [13] . Two endogenous cysteines (C214 and C331) in KCNQ1 were removed to prevent fluorescence labelling of these two cysteines [13] . Mutations were introduced using Quikchange site-directed mutagenesis kit (Qiagen) and fully sequenced to ensure incorporation of intended mutations and the absence of unwanted mutations (sequencing by Genewiz). In vitro transcription of cRNA was performed using mMessage mMachine T7 RNA Transcription Kit (Ambion). VCF recordings Twenty-five nanograms of KCNQ1 RNA with 8 ng of KCNE1 RNA were injected into defolliculated Xenopus laevis oocytes. VCF experiments were performed 2–5 days after injection. Oocytes were labelled for 30 min with 100 μM Alexa488 maleimide or tetramethylrhodamine-5-maleimide (Molecular Probes) in regular ND96 solution (in mM: 96 NaCl, 2 KCl, 1.8 CaCl 2 , 1 MgCl 2 and 5 HEPES, pH 7.5, with NaOH) at 4 °C. Following labelling, they were kept on ice to prevent internalization of labelled channels. Oocytes were placed into a recording chamber in ND96 solution. We used 100 μM LaCl 3 to block endogenous hyperpolarization activated currents. In UCL 2077 and chromanol 293B experiments, 10 μM of the blocker was perfused into the bath at 1 ml min −1 . VCF experiments were carried out as previously reported [26] . Vaseline-gap cut-open voltage clamp electrophysiology Gating currents from KCNQ1/KCNE1 channels were measured using a DAGAN CA-1B cut-open oocyte voltage clamp amplifier (Dagan Corporation, MN, USA) [34] . The composition of the external and internal solutions were respectively (in mM): 100 tetraethylammonium-hydroxide (TEA-OH), 2 Ca(OH) 2 , and 10 HEPES and 100 TEA-OH, 1 ethylene glycol tetraacetic acid and 10 HEPES, both adjusted to pH 7.5 with methane sulphonic acid (MES acid). Oocytes were permeabilized in the lower chamber with 0.3% saponin (with the internal solution) for 30 s. In order to deplete intracellular K + , oocytes were held at 0 mV for 30 min in a solution containing (in mM): 100 N-methyl-D-glucamine, 4 Ca(OH) 2 and 10 HEPES, pH 7.5, adjusted with MES acid. Thereafter, the cells were exposed to the external solution and oocytes were held at −80 mV and prepulse to −140 mV for 3 s before stepping to potentials between −60 and +80 mV of 500 ms duration in 20 mV intervals, followed by a final pulse of −100 mV for 500 ms. Microelectrodes of borosilicate glass capillary tubes had a resistance of 0.3–0.5 MΩ when filled with 3 M Cs-MES and 25 mM CsCl. Data were filtered at 2 kHz and sampled at 50 kHz using the Axon Digidata 1320A (Axon Instruments) collected using Clampex 10.2 (Axon Instruments). MTSET modification We assayed external accessibility with bath perfusion of oocytes under two-electrode voltage clamp (TEVC). The inserted cysteines in KCNQ1 were covalently modified by the membrane-impermeant thiol reagent MTSET (2-(Trimethylammonium)ethyl]methanethiosulfonate Bromide) (Toronto Research Chemicals, Downsview, ON, Canada). A 1–100-mM stock solution of MTSET dissolved in distilled water was stored on ice and was used to provide aliquots that were freshly diluted in regular ND96 solution ~30 s before perfusion. Currents were recorded using a Dagan CA-1B amplifier, low-pass filtered at 1 kHz and sampled at 5 kHz. Microelectrodes had a resistance of 0.3–0.5 MΩ when filled with 3 M KCl. The rate of modification was measured by plotting the change in the current by the MTS reagent as a function of the exposure to the MTSET reagents (exposure=concentration × time, measured in (M s)) and fitted with an exponential (I (exposure) =I 0 exp(−exposure/ τ) . From the τ values (in M s), we calculate the second order rate constants, 1 /τ=k open (M −1 s −1 ) of the MTS reaction. Modelling Fluorescence and currents from the KCNQ1/KCNE1 models were simulated using Berkeley Madonna (Berkeley, CA, USA). Rate constants for each transitions were of the form k i (V)=k i (V i ) × exp (z i F(V-V i )/RT) , where k i (V i ) and z i were determined from data in Fig. 6 ( Supplementary Table 1 ). R , T and F have their usual thermodynamic meaning. Data analysis The steady-state voltage dependence of the current was measured from exponential fits of tail currents following different test potentials. For experiments in ND96 solution, tail currents are measured at −40 mV following 5 s test pulses to voltages between −180 and +100 mV. For experiments in high K + solution, tail currents are measured at −140 mV following 2 s test pulses to voltages between −140 mV and +80 mV. The fit of the tails were extrapolated to the beginning of the tail pulse. Each G(V) experiment was fit with a Boltzmann equation: where A 0 and A 1 are the minimum and maximum, respectively, V 1/2 the voltage at which there is half-maximal activation and K is the slope. Data were normalized between the A 0 and A 1 values of the fit. Fluorescence signals were bleach-subtracted and data points were averaged over tens of milliseconds at the end of the test pulse to reduce errors from signal noise. Fluorescence data is fit with a sum of two Boltzmann distributions and normalized between A 0 and A 2 parameters for each experiment For experiment where the fluorescence did not clearly saturate in the experimental voltage range (such as for K70N), this normalization is an approximation. How to cite this article: Barro-Soria, R. et al. KCNE1 divides the voltage sensor movement in KCNQ1/KCNE1 channels into two steps. Nat. Commun. 5:3750 doi: 10.1038/ncomms4750 (2014).